Smad6-specific recruitment of Smurf E3 ligases mediates TGF-β1-induced degradation of MyD88 in TLR4 signalling Transforming growth factor-β (TGF-β) is a potent anti-inflammatory cytokine that regulates interleukin-1 receptor and Toll-like receptor (TLR) signalling. Here we show a novel mechanism where TGF-β1-induced K48-linked polyubiquitination and degradation of the adaptor MyD88 protein is dependent on the Smad6 protein, but not Smad7, and mediated by recruitment of the Smad ubiquitin regulator factor proteins, Smurf1 and Smurf2, which have E3-ubiquitin ligase activity. Smurf1 interaction with MyD88 appears to be mediated by Smad6, and Smurf2 interaction by Smurf1. Knockdown of endogenous Smurf1 or Smurf2 by RNA interference significantly suppresses the anti-inflammatory effects of TGF-β1 by preventing lipopolysaccharide-induced NF-κB nuclear translocation, resulting in de-suppression of pro-inflammatory gene expression. Similar effects are observed on the lipoteichoic-acid-induced TLR2 pathway, which is also MyD88-dependent, but not the MyD88-independent TLR3 pathway. Thus, our results suggest that MyD88 degradation driven by the Smad6–Smurf pathway is a novel mechanism for TGF-β1-mediated negative regulation of MyD88-dependent pro-inflammatory signalling. Transforming growth factor-β (TGF-β) is a cytokine important in immune system regulation [1] , [2] . TGF-β has a pivotal role in anti-inflammatory cellular responses where the inhibitory Smads (I-Smads), Smad6 and Smad7, act as important mediators by negatively regulating interleukin-1 receptor/Toll-like receptor (IL-1R/TLR) and tumor necrosis factor-alpha (TNF-α) signals [3] , [4] , [5] . I-Smads were originally identified as antagonist proteins of TGF-β/bone morphogenic protein signalling that recruit the HECT E3 ubiquitin ligases Smad ubiquitin regulatory factor 1 (Smurf1) and Smurf2 (refs 6 , 7 , 8 , 9 , 10 , 11 ), and accumulating evidence indicates that the I-Smads also have roles mediating cross-talk between TGF-β and other signalling pathways [4] , [5] , [12] , [13] , [14] . IL-1R and TLR share a conserved cytoplasmic Toll/IL-1R (TIR) domain and downstream signalling complexes, and activation leads to inflammatory response amplification and innate immune response initiation [15] , [16] , [17] , [18] . IL-1R/TLR receptor-mediated signalling is divided into largely two pathways; the myeloid differentiation factor 88 (MyD88)-dependent and -independent pathways [17] , [18] . MyD88 is a cytosolic adaptor protein with a TIR domain at its C-terminal that can associate with the IL-1R/TLR cytoplasmic TIR domain and mediate the formation of signalling complexes [17] , [18] , [19] , [20] . When ligand binding occurs, the interaction between the TIR domains of IL-1R/TLR and MyD88 transmits the signal to interleukin-1 receptor associated kinase (IRAK), subsequently activating the transcription factors NF-κB and AP-1 to increase pro-inflammatory gene expression [17] , [21] . In pathological conditions, the dysregulation of the IL-1R/TLR pro-inflammatory signal may be a major reason for symptoms including septic shock [22] , bone destruction [23] and asthma [24] . Molecular mechanisms underlying the negative regulation of IL-1R/TLR signalling in innate immunity and inflammatory responses have been discovered to be exerted by distinct proteins such as IL-1RII (ref. 25 ), SIGIRR (ref. 26 ), ST2 (ref. 27 ), IRAK-M (ref. 28 ), a MyD88 splice variant (ref. 29 ), and SOCS-1 (ref. 30 ). In addition, the anti-inflammatory cytokine TGF-β1 is responsible for negative regulation of IL-1R/TLR signalling [4] . TGF-β1-induced Smad6 suppresses IL-1R/TLR signalling through direct binding with the adaptor protein Pellino-1, and thus mediates TGF-β-induced anti-inflammation [4] . TGF-β1 also facilitates the ubiquitination and proteasomal degradation of MyD88, subsequently inhibiting lipopolysaccharide (LPS)-induced TLR4 signalling [3] . Therefore, it appears that TGF-β1 augments its anti-inflammatory activity at multiple levels by targeting Pellino-1 and MyD88. However, the molecular mechanism by which MyD88 is ubiquitinated and degraded by TGF-β1 is unknown. Here we demonstrate that TGF-β1-induced ubiquitination and degradation of MyD88 is mediated by Smad6 via recruitment of Smurf proteins, but not by Smad7, suggesting a new mechanism for TGF-β1 mediated inhibition of pro-inflammatory signalling. Smad6 is involved in TGF-β1-induced MyD88 degradation We hypothesized that the inhibitory Smads, Smad6 and Smad7, may be involved in TGF-β1-induced MyD88 degradation, because I-Smads are known to recruit the Smurf E3 ubiquitin ligase proteins [6] , [9] , [10] . The ubiquitination and degradation of endogenous MyD88 protein in SMAD6 knockdown or SMAD7 knockdown primary peritoneal macrophages was examined to determine whether the I-Smads are involved in regulation of MyD88 levels. Mutant Serpinb2 -specific short interfering RNA (si-mPAI-2) was used as a negative control for lentivirus infection [4] . MyD88 was ubiquitinated and subsequently degraded in TGF-β1-treated SMAD7 knockdown primary peritoneal macrophages and CMT-93 mouse epithelial cells ( Fig. 1a , lane 9,10; Supplementary Fig. S1 ). In contrast, ubiquitination levels of endogenous MyD88 protein did not increase, and MyD88 was not degraded on TGF-β1 treatment in primary macrophages with SMAD6 knocked-down using multiple independent SMAD6-specific siRNAs, as well as in SMAD6 knockdown CMT-93 cells ( Fig. 1a , lane 3–8; Supplementary Fig. S1 ). To exclude nonspecific binding to ubiquitin, cell lysates were prepared in lysis buffer containing 1% SDS and membranes containing SDS–PAGE-separated immunoprecipitates were treated with denaturation buffer containing 6 M guanidine chloride. To confirm these results, ubiquitination and degradation of Flag-MyD88 was examined in SMAD6 wild type or SMAD6 knockdown CMT-93 cells co-transfected with Flag-MyD88 and His-ubiquitin ( Fig. 1b ). MyD88 ubiquitination and degradation increased on TGF-β1 treatment in a time-dependent manner in SMAD6 -expressing CMT-93 cells, but not in SMAD6 knockdown cells ( Fig. 1b ). These phenomena were also observed in pull-down experiments using Ni-NTA agarose ( Fig. 1c ). In addition, TGF-β1-induced ubiquitination and degradation of MyD88 decreased after 6 h of TGF-β1 treatment and showed a correlation with changes in Smad6 expression ( Fig. 1d ). TGF-β1-induced degradation of MyD88 was inhibited by the proteasomal inhibitor MG132 ( Fig. 1e ). These results indicate that TGF-β1-induced MyD88 ubiquitination and degradation is dependent on Smad6, but not Smad7. 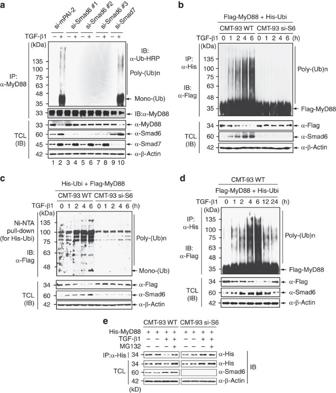Figure 1: TGF-β1-induced MyD88 ubiquitination and degradation requires the Smad6 and Smurf proteins. (a) Primary peritoneal macrophages were infected with lentiviruses expressingSMAD6- orSMAD7-specific siRNAs and treated for 6 h with 5 ng ml−1TGF-β1. A lentivirus expressing mutantSerpinb2-specific siRNA (si-mPAI-2) was used as a negative control4. Ubiquitination levels of endogenous MyD88 were observed by immunoprecipitation (IP) with anti-MyD88 antibody and immunoblotting (IB) with anti-ubiquitin-HRP. (b) Flag-MyD88 ubiquitination and degradation was examined inSMAD6WT orSMAD6knockdown (si-S6) CMT-93 cells co-transfected with Flag-MyD88 and His-ubiquitin (His-Ubi). (c)SMAD6knockdown CMT-93 cells (CMT-93-si-S6) or wild-type CMT-93 cells (CMT-93-WT) were transfected with Flag-MyD88 and His-Ubi plasmids, and treated with TGF-β1. Flag-MyD88 ubiquitination was examined by pull-down assays using Ni-NTA agarose, followed by immunoblotting with anti-Flag antibody. Endogenous Smad6 was detected with anti-Smad6 antibody. (d) To examine TGF-β1-induced MyD88 ubiquitination and degradation after 6 h of TGF-β1 treatment,SMAD6-expressing CMT-93 wild type (WT) cells were co-transfected with Flag-MyD88 and His-Ubi. (e) TGF-β1-induced MyD88 degradation was inhibited by the proteasomal inhibitor MG132. His-MyD88 was co-transfected intoSMAD6WT orSMAD6knockdown (si-S6) CMT-93 cells. Cells were pre-treated with MG132 for 6 h, followed by TGF-β1 treatment for 6 h. For (b,d), Flag-MyD88 ubiquitination was observed by immunoprecipitation with anti-His antibody and immunoblotting with anti-Flag antibody. Expression of the β-actin protein was used as a loading control. All data are representative of at least three independent experiments. TCL, total cell lysates; WT, wild type. Figure 1: TGF-β1-induced MyD88 ubiquitination and degradation requires the Smad6 and Smurf proteins. ( a ) Primary peritoneal macrophages were infected with lentiviruses expressing SMAD6 - or SMAD7 -specific siRNAs and treated for 6 h with 5 ng ml −1 TGF-β1. A lentivirus expressing mutant Serpinb2 -specific siRNA (si-mPAI-2) was used as a negative control [4] . Ubiquitination levels of endogenous MyD88 were observed by immunoprecipitation (IP) with anti-MyD88 antibody and immunoblotting (IB) with anti-ubiquitin-HRP. ( b ) Flag-MyD88 ubiquitination and degradation was examined in SMAD6 WT or SMAD6 knockdown (si-S6) CMT-93 cells co-transfected with Flag-MyD88 and His-ubiquitin (His-Ubi). ( c ) SMAD6 knockdown CMT-93 cells (CMT-93-si-S6) or wild-type CMT-93 cells (CMT-93-WT) were transfected with Flag-MyD88 and His-Ubi plasmids, and treated with TGF-β1. Flag-MyD88 ubiquitination was examined by pull-down assays using Ni-NTA agarose, followed by immunoblotting with anti-Flag antibody. Endogenous Smad6 was detected with anti-Smad6 antibody. ( d ) To examine TGF-β1-induced MyD88 ubiquitination and degradation after 6 h of TGF-β1 treatment, SMAD6 -expressing CMT-93 wild type (WT) cells were co-transfected with Flag-MyD88 and His-Ubi. ( e ) TGF-β1-induced MyD88 degradation was inhibited by the proteasomal inhibitor MG132. His-MyD88 was co-transfected into SMAD6 WT or SMAD6 knockdown (si-S6) CMT-93 cells. Cells were pre-treated with MG132 for 6 h, followed by TGF-β1 treatment for 6 h. For ( b , d ), Flag-MyD88 ubiquitination was observed by immunoprecipitation with anti-His antibody and immunoblotting with anti-Flag antibody. Expression of the β-actin protein was used as a loading control. All data are representative of at least three independent experiments. TCL, total cell lysates; WT, wild type. Full size image Smurf proteins ubiquitinate MyD88 protein for degradation Many E3 ubiquitin ligases have critical roles in target protein recognition and degradation by the 26S proteasomes in the TGF-β signalling pathway [31] . We tested whether the HECT E3 ubiquitin ligases Smurf1 and Smurf2, known to interact with the I-Smads, have roles in regulation of MyD88 protein levels. The ubiquitination and degradation of endogenous MyD88 protein was blocked in SMURF1 or SMURF2 knockdown primary peritoneal macrophages and CMT-93 cells treated with TGF-β1, even though endogenous Smad6 expression was increased ( Fig. 2a ; Supplementary Fig. S2 ). Two independent siRNAs each were used to generate SMURF1 - or SMURF2 -specific knockdown primary peritoneal macrophages. In addition, overexpression of Myc-tagged Smurf1 or HA-tagged Smurf2 further increased the ubiquitination levels of MyD88 in the presence of Smad6 ( Fig. 2b , lane 3,5). Consistently, site-directed mutants of Smurf1 (C699A) and Smurf2 (C695A), where cysteine residues important for E3 ubiquitin ligase activity were mutated into alanines, did not induce TGF-β1-mediated ubiquitination and degradation of MyD88 ( Fig. 2b , lane 4,6). These results indicate that both Smurf1 and Smurf2 are required for negative regulation of the MyD88 protein by ubiquitination. 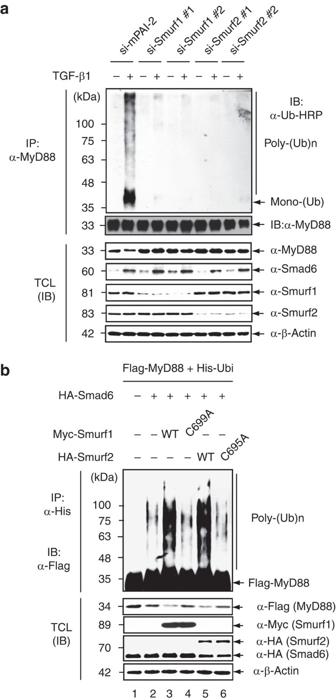Figure 2: Smurf proteins are required for TGF-β1-induced MyD88 ubiquitination and degradation. (a) Primary peritoneal macrophages were infected with lentiviruses expressingSMURF1- (si-Smurf1) orSMURF2-specific (si-Smurf2) siRNAs and treated with 5 ng ml−1TGF-β1 for 6 h. A lentivirus expressing mutantSerpinb2-specific siRNA (si-mPAI-2) was used as a negative control4. Ubiquitination levels of endogenous MyD88 were observed by immunoprecipitation (IP) with anti-MyD88 antibody and immunoblotting (IB) with anti-ubiquitin-HRP. (b) Overexpression of Myc-Smurf1 or HA-Smurf2 increases Flag-MyD88 ubiquitination. HA-Smad6, Myc-Smurf1(WT), Myc-Smurf1(C699A), HA-Smurf2(WT), and HA-Smurf2(C695A) were co-transfected with Flag-MyD88 and His-Ubi in the indicated combinations into CMT-93 cells. Flag-MyD88 ubiquitination was observed by immunoprecipitation with anti-His antibody and immunoblotting with anti-Flag antibody. Expression of the β-actin protein was used as a loading control. All data are representative of at least three independent experiments. TCL, total cell lysates; WT, wild type. Figure 2: Smurf proteins are required for TGF-β1-induced MyD88 ubiquitination and degradation. ( a ) Primary peritoneal macrophages were infected with lentiviruses expressing SMURF1 - (si-Smurf1) or SMURF2 -specific (si-Smurf2) siRNAs and treated with 5 ng ml −1 TGF-β1 for 6 h. A lentivirus expressing mutant Serpinb2 -specific siRNA (si-mPAI-2) was used as a negative control [4] . Ubiquitination levels of endogenous MyD88 were observed by immunoprecipitation (IP) with anti-MyD88 antibody and immunoblotting (IB) with anti-ubiquitin-HRP. ( b ) Overexpression of Myc-Smurf1 or HA-Smurf2 increases Flag-MyD88 ubiquitination. HA-Smad6, Myc-Smurf1(WT), Myc-Smurf1(C699A), HA-Smurf2(WT), and HA-Smurf2(C695A) were co-transfected with Flag-MyD88 and His-Ubi in the indicated combinations into CMT-93 cells. Flag-MyD88 ubiquitination was observed by immunoprecipitation with anti-His antibody and immunoblotting with anti-Flag antibody. Expression of the β-actin protein was used as a loading control. All data are representative of at least three independent experiments. TCL, total cell lysates; WT, wild type. Full size image Smurf1 is recruited to MyD88 through interaction with Smad6 Next, physical interactions between the Smad6, MyD88 and Smurf proteins were tested. Plasmids encoding His-tagged MyD88, Myc-Smurf1, Flag-Smurf2, or HA-Smad6 were transiently transfected in various combinations into CMT-93 cells, and immunoprecipitations were performed with the indicated antibodies. Experiments were done with MG132 pre-treatment, to prevent MyD88 degradation by TGF-β1-induced Smad6, and promote visualization. MyD88 protein interacted with both Smad6 and Smurf1, but not Smurf2 ( Fig. 3a , lanes 1,2,3), whereas Smad6 bound to Smurf1, but not Smurf2 ( Fig. 3a , lanes 4,5). These results indicate that MyD88, Smad6 and Smurf1 physically interact. Smurf2 was observed to only bind to Smurf1 ( Fig. 3a , lane 6), as reported [32] , suggesting that Smurf2 is involved in MyD88 degradation through interaction with Smurf1. This interaction between the MyD88, Smad6 and Smurf1 proteins was confirmed by immunoprecipitation against endogenous proteins in TGF-β1-treated primary peritoneal macrophages ( Fig. 3b , lanes 1,2). The interaction between MyD88 and Smurf1 was abolished by SMAD6 knockdown in peritoneal macrophage cells and CMT-93 cells ( Fig. 3b , lanes 3,4; Fig. 3c , lane 1), and ectopic expression of Smad6 in SMAD6 knockdown CMT-93 cells restored the interaction ( Fig. 3c , lane 4). The Smurf1–Smurf2 interaction was still observed in SMAD6 knockdown cells ( Fig. 3c , lane 3). A basal interaction between Smad6 and MyD88 was observed even in the absence of TGF-β1 ( Fig. 3b ; lane 1), which is probably caused by the 3% thioglycollate injection used in the preparation of primary peritoneal macrophages. Injection of thioglycollate appears to slightly increase expression of the Smad6 gene [4] , resulting in this basal interaction even in the absence of TGF-β1. Consistent with our results, immunofluorescence experiments also showed co-localization of ectopically expressed MyD88, Smad6 and Smurf1, mainly in the cytoplasm of CMT-93 wild-type cells ( Fig. 3d ). These results revealed that Smurf1 is recruited to MyD88 through direct interaction with Smad6. 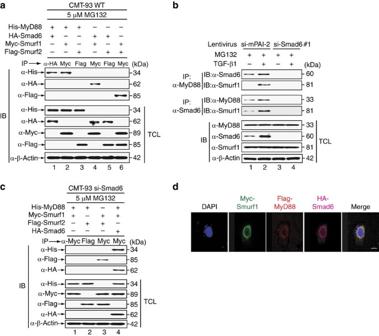Figure 3: Recruitment of Smurf1 to MyD88 is dependent on Smad6. (a) Interactions between the MyD88, Smad6, Smurf1, and Smurf2 proteins. Indicated plasmids were co-transfected into CMT-93 cells. IP and IB were performed with the indicated antibodies. TCL; total cell lysates. (b) Primary peritoneal macrophages were infected with lentiviruses expressingSMAD6-specific siRNA (si-Smad6 #1) or mutantSerpinb2-specific siRNA (si-mPAI-2). Cells were pre-treated with the proteasome inhibitor MG132 for 6 h, and then treated with TGF-β1 for 2 h. To confirm the interaction of endogenous MyD88, Smad6, and Smurf1 proteins, IP and IB were performed with the indicated antibodies to endogenous proteins. (c) Ectopic expression of Smad6 inSMAD6knockdown CMT-93 cells restores the interaction between MyD88 and Smurf1. IP and IB were performed with the indicated antibodies. (d) Immunofluorescent staining of Myc-Smurf1, Flag-MyD88, and HA-Smad6 in CMT-93 cells show co-localization. Nuclei were stained with DAPI. Scale bar, 10 μm. All data are representative of at least three independent experiments. Figure 3: Recruitment of Smurf1 to MyD88 is dependent on Smad6. ( a ) Interactions between the MyD88, Smad6, Smurf1, and Smurf2 proteins. Indicated plasmids were co-transfected into CMT-93 cells. IP and IB were performed with the indicated antibodies. TCL; total cell lysates. ( b ) Primary peritoneal macrophages were infected with lentiviruses expressing SMAD6 -specific siRNA (si-Smad6 #1) or mutant Serpinb2 -specific siRNA (si-mPAI-2). Cells were pre-treated with the proteasome inhibitor MG132 for 6 h, and then treated with TGF-β1 for 2 h. To confirm the interaction of endogenous MyD88, Smad6, and Smurf1 proteins, IP and IB were performed with the indicated antibodies to endogenous proteins. ( c ) Ectopic expression of Smad6 in SMAD6 knockdown CMT-93 cells restores the interaction between MyD88 and Smurf1. IP and IB were performed with the indicated antibodies. ( d ) Immunofluorescent staining of Myc-Smurf1, Flag-MyD88, and HA-Smad6 in CMT-93 cells show co-localization. Nuclei were stained with DAPI. Scale bar, 10 μm. All data are representative of at least three independent experiments. Full size image Distinct domains of Smad6 bind to MyD88 and Smurf1 Next, we tested which domains of Smad6 participate in the interactions with MyD88 and Smurf1. Three truncated mutants of Smad6 containing the MH1-like, Linker or MH2 domain [33] ( Fig. 4a ), respectively, were co-transfected into HEK293 cells with full-length His-MyD88 or Myc-Smurf1 ( Fig. 4b,c ). HEK293 cells were used in these experiments because HEK293 cells express SMAD6 at very low levels and do not respond to TGF-β1. Coimmunoprecipitation analysis showed that the Smad6 MH1-like domain (amino acids 1–180) specifically binds to MyD88, and the Linker domain (amino acids 181–331) interacts with Smurf1 ( Fig. 4b,c ). To find the regions of MyD88 that bind to Smad6, the MyD88 protein was divided into three regions (N, M and C regions) ( Fig. 4d ). Coimmunoprecipitation assays in HEK293 cells with HA-Smad6 showeded that amino acids 201–297 (C region) of MyD88 are sufficient for interaction with Smad6 ( Fig. 4e ). These results demonstrate that MyD88–Smad6 interaction is mediated by the direct interaction between the C region of MyD88 and MH1-like region of Smad6. We re-confirmed that Smad6 is necessary for the interaction between MyD88 and Smurf1 by looking at the interaction between the MyD88 C region and Smurf1 in SMAD6 knockdown and wild-type CMT-93 cells ( Fig. 4f ). The interaction between the MyD88 C region and Smurf1 was not observed in SMAD6 knockdown cells ( Fig. 4f ). 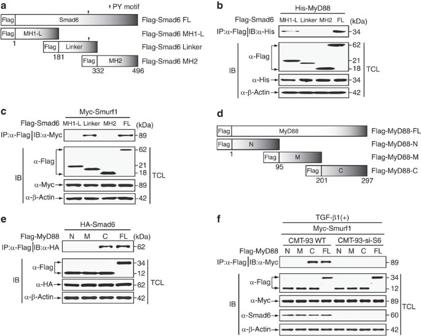Figure 4: Smad6 interacts with MyD88 and Smurf1 through different domains. (a) Schematic representation of the truncated Smad6 mutants33. (b) Truncated Smad6 mutants were co-transfected with the His-tagged full length MyD88 plasmid into HEK293 cells. Cell lysates were immunoprecipitated with anti-Flag antibody and immunoblotted with anti-His antibody. TCL; total cell lysates. (c) Truncated Smad6 mutants were co-transfected with the Myc-tagged full-length Smurf1 plasmid into HEK293 cells. Cell lysates were immunoprecipitated with anti-Flag antibody and immunoblotted with anti-Myc antibody. (d) Schematic representation of plasmids encoding different truncated forms of MyD88. (e) Truncated mutants of MyD88 were co-transfected with the HA-tagged full-length Smad6 plasmid into HEK293 cells. Cell lysates were immunoprecipitated with anti-Flag antibody and immunoblotted with anti-HA antibody. (f) Smad6 is necessary for the interaction between the MyD88 C region and Smurf1. Truncated mutants of MyD88 were co-transfected with the Myc-Smurf1 plasmid intoSMAD6-WT orSMAD6knockdown CMT-93 cells. Cells were pre-treated with 5 μM MG132 followed by TGF-β1 treatment for 2 h, and cell lysates were immunoprecipitated with anti-Flag antibody and immunoblotted with anti-Myc antibody. All data are representative of at least three independent experiments. Figure 4: Smad6 interacts with MyD88 and Smurf1 through different domains. ( a ) Schematic representation of the truncated Smad6 mutants [33] . ( b ) Truncated Smad6 mutants were co-transfected with the His-tagged full length MyD88 plasmid into HEK293 cells. Cell lysates were immunoprecipitated with anti-Flag antibody and immunoblotted with anti-His antibody. TCL; total cell lysates. ( c ) Truncated Smad6 mutants were co-transfected with the Myc-tagged full-length Smurf1 plasmid into HEK293 cells. Cell lysates were immunoprecipitated with anti-Flag antibody and immunoblotted with anti-Myc antibody. ( d ) Schematic representation of plasmids encoding different truncated forms of MyD88. ( e ) Truncated mutants of MyD88 were co-transfected with the HA-tagged full-length Smad6 plasmid into HEK293 cells. Cell lysates were immunoprecipitated with anti-Flag antibody and immunoblotted with anti-HA antibody. ( f ) Smad6 is necessary for the interaction between the MyD88 C region and Smurf1. Truncated mutants of MyD88 were co-transfected with the Myc-Smurf1 plasmid into SMAD6 -WT or SMAD6 knockdown CMT-93 cells. Cells were pre-treated with 5 μM MG132 followed by TGF-β1 treatment for 2 h, and cell lysates were immunoprecipitated with anti-Flag antibody and immunoblotted with anti-Myc antibody. All data are representative of at least three independent experiments. Full size image MyD88 lysine 231 and 262 are polyubiquitinated by TGF-β1 The MyD88 protein has 15 lysine residues as possible sites for polyubiquitination. To determine which lysine residues are critical in TGF-β1-induced MyD88 ubiquitination, full-length MyD88 was divided into two regions, L and R ( Fig. 5a ). These plasmids were co-transfected into CMT-93 wild type cells with the His-Ubi plasmid and cells were treated with TGF-β1. The R region of MyD88, which contains 11 lysine residues, was ubiquitinated and degraded on TGF-β1 treatment, but the L region was not ( Fig. 5b ). To determine which lysine residues in the R region are involved in MyD88 ubiquitination, each lysine residue was substituted with arginine, and ubiquitination of each mutant protein was examined in SMAD6 -expressing CMT-93 cells. Among the 11 mutants, K231R and K262R, where the lysine residues 231 and 262 were mutated into arginines, respectively, were resistant to TGF-β1-induced ubiquitination and degradation ( Fig. 5c ). Next, to determine whether lysine 48-linked or lysine 63-linked polyubiquitin chains are formed on MyD88 on TGF-β1 treatment, mutant plasmids encoding ubiquitin with six lysine residues mutated to alanines, except for lysine residue 48 (His-Ubi-K48), or with six lysine residues mutated to alanines, except for lysine residue 63 (His-Ubi-K63), were transfected into CMT-93 cells. Plasmids encoding His-tagged wild-type ubiquitin (His-Ubi) and His-Ubi-7KR with seven lysine residues mutated to alanines were used as controls. Immunoprecipitation assays, following 6 h of TGF-β1 treatment, showed that TGF-β1 induces MyD88 degradation through the K48-linked polyubiquitination of MyD88 ( Fig. 5d ). Next, to examine whether TGF-β1-induced ubiquitination of MyD88 lysine residues 231 and 262 are important for TGF-β1-mediated negative regulation of MyD88-dependent TLR4 signalling, we generated MYD88 knockdown CMT-93 cells, into which a 5× NF-κB-Luc reporter plasmid was co-transfected with a plasmid encoding Flag-MyD88 K231/261R, which is resistant to TGF-β1-induced degradation. We predicted that expression of Flag-MyD88 K231/262R in MYD88 -depleted cells would prevent inhibition of LPS-induced NF-κB activation by TGF-β1 treatment. However, we did not observe changes in NF-κB activity on treatment of TGF-β1 ( Supplementary Fig. S3 ). The K231/261R double mutant, with lysine residues 231 and 262 both mutated into arginines, could not induce LPS-mediated NF-κB activation in MYD88 -depleted cells even in the absence of TGF-β1. It is possible that mutations in both lysine residues 231 and 262 affect the intrinsic function of MyD88 involved in TLR4 signalling. 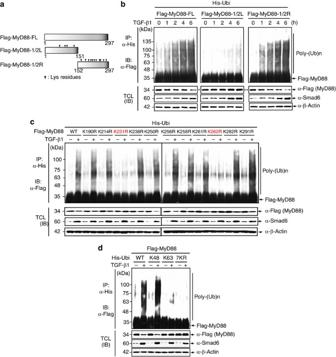Figure 5: The MyD88 lysine residues 231 and 262 are sites of TGF-β1-induced K48-linked polyubiquitination. (a) Schematic representation of the truncated MyD88 mutants, Flag-MyD88-1/2L and Flag-MyD88-1/2R. (b) Plasmids encoding full-length MyD88 (Flag-MyD88-FL) and the truncated 1/2L and 1/2R mutants were transfected into CMT-93 cells with a plasmid encoding His-Ubi. Cells were treated with TGF-β1 for the indicated time periods. IP and IB were performed with the indicated antibodies. (c) Plasmids encoding point mutants where the indicated lysine residue is substituted with arginine were co-transfected into CMT-93 cells with the His-Ubi plasmid. All cells were treated with TGF-β1 for 6 h. IP and IB were performed with the indicated antibodies. (d) A plasmid encoding a wild-type (WT) ubiquitin protein (HA-Ubi) or ubiquitin mutants that only mediate K48-linked (HA-Ubi-K48) or K63-linked (HA-Ubi-K63) polyubiquitination were transfected into CMT-93 cells with Flag-MyD88 and treated with TGF-β1 for 6 h. Seven lysine residues of ubiquitin were mutated to arginines in His-Ubi7KR. IP and IB were performed with the indicated antibodies. All data are representative of at least three independent experiments. Figure 5: The MyD88 lysine residues 231 and 262 are sites of TGF-β1-induced K48-linked polyubiquitination. ( a ) Schematic representation of the truncated MyD88 mutants, Flag-MyD88-1/2L and Flag-MyD88-1/2R. ( b ) Plasmids encoding full-length MyD88 (Flag-MyD88-FL) and the truncated 1/2L and 1/2R mutants were transfected into CMT-93 cells with a plasmid encoding His-Ubi. Cells were treated with TGF-β1 for the indicated time periods. IP and IB were performed with the indicated antibodies. ( c ) Plasmids encoding point mutants where the indicated lysine residue is substituted with arginine were co-transfected into CMT-93 cells with the His-Ubi plasmid. All cells were treated with TGF-β1 for 6 h. IP and IB were performed with the indicated antibodies. ( d ) A plasmid encoding a wild-type (WT) ubiquitin protein (HA-Ubi) or ubiquitin mutants that only mediate K48-linked (HA-Ubi-K48) or K63-linked (HA-Ubi-K63) polyubiquitination were transfected into CMT-93 cells with Flag-MyD88 and treated with TGF-β1 for 6 h. Seven lysine residues of ubiquitin were mutated to arginines in His-Ubi7KR. IP and IB were performed with the indicated antibodies. All data are representative of at least three independent experiments. Full size image Smurf proteins inhibit LPS-induced NF-κB activity As activity of the transcription factor NF-κB is inhibited by TGF-β1 signalling, we tested whether Smurf1 and Smurf2 are involved in this inhibition by examining the nuclear translocation of NF-κB in SMURF1 or SMURF2 knockdown CMT-93 cells. In CMT-93 wild-type cells (CMT-93-si-mPAI-2), LPS treatment resulted in nuclear translocation of NF-κB, which was inhibited by TGF-β1 pre-treatment ( Fig. 6a ). However, in SMURF1 or SMURF2 knockdown CMT-93 cells, TGF-β1 pre-treatment could not inhibit LPS-induced nuclear translocation of NF-κB ( Fig. 6b,c ). SMAD6 knockdown CMT-93 cells also showed similar results to the SMURF knockdown CMT-93 cells ( Fig. 6d ), indicating that the Smurf proteins, as well as Smad6, are involved in TGF-β1-induced inhibition of NF-κB nuclear translocation. 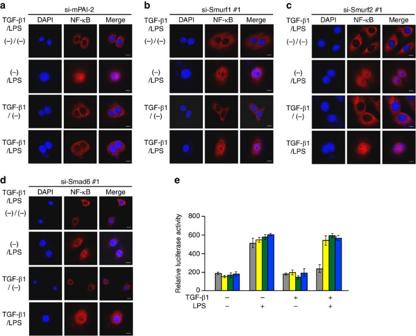Figure 6: Knockdown ofSMURF1orSMURF2blocks TGF-β1-induced inhibition of NF-κB nuclear translocation. (a) Fluorescence microscopy of CMT-93 cells infected with lentiviruses expressing mutantSerpinb2siRNA (si-mPAI-2) as a negative control. Scale bar, 10 μm. (b) Fluorescence microscopy of CMT-93 cells infected with lentiviruses expressingSMURF1-specific siRNA (si-Smurf1 #1). Scale bar, 10 μm. (c) Fluorescence microscopy of CMT-93 cells infected with lentiviruses expressingSMURF2-specific siRNA (si-Smurf2 #1). Scale bar, 10 μm. (d) Fluorescence microscopy of CMT-93 cells infected with lentiviruses expressingSMAD6-specific siRNA (si-Smad6 #1). Cells in (a–d) were pre-treated, or not, with TGF-β1 for 2 h, and then treated, or not with, LPS for 2 h. Cells were stained with anti-NF-κB p65 (red) and nuclei stained with DAPI (blue). Scale bar 10 μm. All data are representative of at least three independent experiments. (e) RAW264.7 macrophages were infected with lentiviruses expressing different siRNAs. Following 48 h of infection, a 5× NF-κB-Luc reporter plasmid was transfected. Cells were pre-treated with TGF-β1 for 2 h, subsequently treated with LPS for 2 h, and luciferase activities were measured and normalized. Grey bar, si-mPAI-2 expressing cells; yellow bar, si-Smurf1 #1 expressing cells; green bar, si-Smurf2 #1 expressing cells; blue bar, si-Smad6 #1 expressing cells. All data represent the mean±s.d. of three independent experiments. Figure 6: Knockdown of SMURF1 or SMURF2 blocks TGF-β1-induced inhibition of NF-κB nuclear translocation. ( a ) Fluorescence microscopy of CMT-93 cells infected with lentiviruses expressing mutant Serpinb2 siRNA (si-mPAI-2) as a negative control. Scale bar, 10 μm. ( b ) Fluorescence microscopy of CMT-93 cells infected with lentiviruses expressing SMURF1 -specific siRNA (si-Smurf1 #1). Scale bar, 10 μm. ( c ) Fluorescence microscopy of CMT-93 cells infected with lentiviruses expressing SMURF2 -specific siRNA (si-Smurf2 #1). Scale bar, 10 μm. ( d ) Fluorescence microscopy of CMT-93 cells infected with lentiviruses expressing SMAD6 -specific siRNA (si-Smad6 #1). Cells in ( a – d ) were pre-treated, or not, with TGF-β1 for 2 h, and then treated, or not with, LPS for 2 h. Cells were stained with anti-NF-κB p65 (red) and nuclei stained with DAPI (blue). Scale bar 10 μm. All data are representative of at least three independent experiments. ( e ) RAW264.7 macrophages were infected with lentiviruses expressing different siRNAs. Following 48 h of infection, a 5× NF-κB-Luc reporter plasmid was transfected. Cells were pre-treated with TGF-β1 for 2 h, subsequently treated with LPS for 2 h, and luciferase activities were measured and normalized. Grey bar, si-mPAI-2 expressing cells; yellow bar, si-Smurf1 #1 expressing cells; green bar, si-Smurf2 #1 expressing cells; blue bar, si-Smad6 #1 expressing cells. All data represent the mean±s.d. of three independent experiments. Full size image We obtained further evidence that the Smurf proteins are involved in regulating the transcriptional activity of NF-κB. First, the expression of an NF-κB-mediated reporter gene was examined in SMURF1 or SMURF2 knockdown RAW264.7 cells. SMURF1 or SMURF2 knockdown RAW264.7 cells were transiently transfected with a 5× NF-κB-Luc reporter plasmid and pre-treated with TGF-β1, followed by LPS treatment. As expected, TGF-β1 treatment inhibited LPS-induced NF-κB-mediated reporter gene induction in control RAW264.7 cells, but not in RAW264.7 cells expressing SMURF1 -, SMURF2 - or SMAD6 -specific siRNA ( Fig. 6e ). Smurf proteins decrease LPS-induced pro-inflammatory genes Next, the expression of pro-inflammatory NF-κB target genes was examined in SMURF1 or SMURF2 knockdown primary macrophages. SMURF1 or SMURF2 knockdown primary macrophages were pre-treated with TGF-β1 for 2 h and treated with LPS, and expression of LPS-induced pro-inflammatory genes such as IL6 and NOS2 were monitored by quantitative real-time RT–PCR and regular RT–PCR. SMAD6 knockdown, or mutant Serpinb2 (mPAI-2) knockdown primary macrophages were used as a positive or negative control, respectively [4] . As expected, expression of pro-inflammatory genes was increased by LPS treatment, but not inhibited by TGF-β1 in SMURF1 or SMURF2 knockdown primary macrophages ( Fig. 7a,b ; Supplementary Fig. S4 ). This result was further confirmed by monitoring IL-6 production in SMURF1 or SMURF2 knockdown primary peritoneal macrophages ( Fig. 7c ). 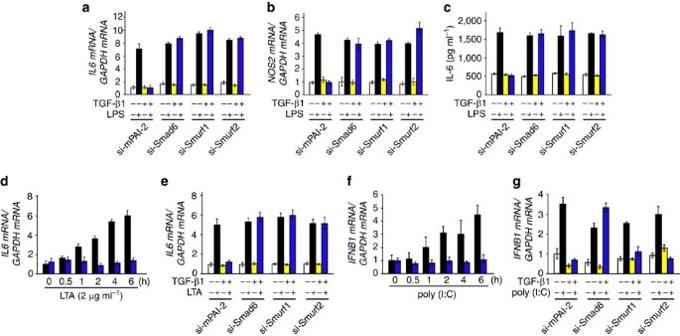Figure 7: Smurf proteins are necessary for the anti-inflammatory activity of TGF-β1. (a,b) NF-κB-mediated pro-inflammatory gene expression was analysed by quantitative real-time RT–PCR. Primary peritoneal macrophages were infected with lentiviruses expressing si-mPAI-2, si-Smurf1 #1, si-Smurf2 #1, or si-Smad6 #1.IL6, interleukin-6;NOS2, inducible nitric oxide synthase-2. (c) ELISA of IL-6 production by primary peritoneal macrophages infected with lentiviruses expressing the indicated siRNAs. For (a), (b) and (c), white bars; no treatment of TGF-β1 or LPS, black bars; LPS treatment for 2 h, yellow bars; TGF-β1 pre-treatment for 2 h, blue bars; TGF-β1 pre-treatment for 2 h and LPS treatment for 2 h. (d)IL6mRNA expression was analysed by quantitative real-time RT–PCR. Primary peritoneal macrophages were not treated (black bars) or pre-treated with TGF-β1 for 2 h (blue bars), and subsequently treated with 2 μg ml−1LTA for the indicated time periods. (e) Expression ofIL6mRNA induced by LTA treatment was analysed in primary peritoneal macrophages infected with lentiviruses expressing the indicated siRNAs by quantitative real-time RT–PCR. White bars, no treatment of TGF-β1 or LTA; black bars, LTA treatment for 6 h; yellow bars, TGF-β1 pre-treatment for 2 h; blue bars, TGF-β1 pre-treatment for 2 h and LTA treatment for 6 h. (f)IFNB1mRNA expression induced by poly (I:C) was analysed by quantitative real-time RT–PCR. Primary peritoneal macrophages were not treated (black bars) or pre-treated with TGF-β1 for 2 h (blue bars), and subsequently treated with 5 μg ml−1poly (I:C) for the indicated time periods. (g)IFNB1mRNA expression induced by 5 μg ml−1poly (I:C) was analysed in primary peritoneal macrophages infected with lentiviruses expressing the indicated siRNAs by quantitative real-time RT–PCR. White bars, no treatment of TGF-β1 or poly (I:C); black bars, poly (I:C) treatment for 6 h; yellow bars, TGF-β1 pre-treatment for 2 h; blue bars, TGF-β1 pre-treatment for 2 h and poly (I:C) treatment for 6 h. All real-time RT–PCR data represent the mean±s.d. of three independent experiments. Figure 7: Smurf proteins are necessary for the anti-inflammatory activity of TGF-β1. ( a , b ) NF-κB-mediated pro-inflammatory gene expression was analysed by quantitative real-time RT–PCR. Primary peritoneal macrophages were infected with lentiviruses expressing si-mPAI-2, si-Smurf1 #1, si-Smurf2 #1, or si-Smad6 #1. IL6 , interleukin-6; NOS2 , inducible nitric oxide synthase-2. ( c ) ELISA of IL-6 production by primary peritoneal macrophages infected with lentiviruses expressing the indicated siRNAs. For ( a ), ( b ) and ( c ), white bars; no treatment of TGF-β1 or LPS, black bars; LPS treatment for 2 h, yellow bars; TGF-β1 pre-treatment for 2 h, blue bars; TGF-β1 pre-treatment for 2 h and LPS treatment for 2 h. ( d ) IL6 mRNA expression was analysed by quantitative real-time RT–PCR. Primary peritoneal macrophages were not treated (black bars) or pre-treated with TGF-β1 for 2 h (blue bars), and subsequently treated with 2 μg ml −1 LTA for the indicated time periods. ( e ) Expression of IL6 mRNA induced by LTA treatment was analysed in primary peritoneal macrophages infected with lentiviruses expressing the indicated siRNAs by quantitative real-time RT–PCR. White bars, no treatment of TGF-β1 or LTA; black bars, LTA treatment for 6 h; yellow bars, TGF-β1 pre-treatment for 2 h; blue bars, TGF-β1 pre-treatment for 2 h and LTA treatment for 6 h. ( f ) IFNB1 mRNA expression induced by poly (I:C) was analysed by quantitative real-time RT–PCR. Primary peritoneal macrophages were not treated (black bars) or pre-treated with TGF-β1 for 2 h (blue bars), and subsequently treated with 5 μg ml −1 poly (I:C) for the indicated time periods. ( g ) IFNB1 mRNA expression induced by 5 μg ml −1 poly (I:C) was analysed in primary peritoneal macrophages infected with lentiviruses expressing the indicated siRNAs by quantitative real-time RT–PCR. White bars, no treatment of TGF-β1 or poly (I:C); black bars, poly (I:C) treatment for 6 h; yellow bars, TGF-β1 pre-treatment for 2 h; blue bars, TGF-β1 pre-treatment for 2 h and poly (I:C) treatment for 6 h. All real-time RT–PCR data represent the mean±s.d. of three independent experiments. Full size image Smurf proteins inhibit MyD88-dependent TLR signalling We hypothesized that TGF-β1 could have anti-inflammatory effects on other MyD88-dependent TLR signalling pathways, in addition to the LPS-induced TLR4 signalling pathway. TLR2 senses various components, such as lipoproteins from bacteria, mycoplasma and fungi, by forming a heterodimer with TLR1 or TLR6 (refs 17 , 34 ). On ligand stimulation, TLR2 induces the production of various pro-inflammatory cytokines such as IL-6 through a MyD88-dependent signalling cascade [34] . Therefore, we hypothesized that TGF-β1 may inhibit TLR2 signalling through MyD88 degradation by the Smad6–Smurf1 pathway. We initially examined whether TGF-β1 can inhibit expression of the lipoteichoic acid (LTA)-induced IL6 gene in primary peritoneal macrophages. The IL6 gene was significantly induced by LTA in a time-dependent manner whereas TGF-β1 pre-treatment for 2 h inhibited expression of the IL6 gene ( Fig. 7d ). Next, we tested whether TGF-β1 inhibition of LTA-induced IL6 gene expression could be suppressed by knockdown of SMAD6 , SMURF1 or SMURF2 in primary peritoneal macrophages The inhibitory effect of TGF-β1 on LTA-induced IL6 gene expression was suppressed in SMAD6 , SMURF1 or SMURF2 knockdown primary peritoneal macrophages compared with the negative control ( Fig. 7e ; Supplementary Fig. S5 ). In contrast, MyD88-independent TLR3 signalling triggered by poly (I:C) was unaffected in SMURF1 or SMURF2 knockdown primary peritoneal macrophages in the presence of TGF-β1 ( Fig. 7f,g ; Supplementary Figs. S6 and S7 ). Interestingly, although it had been reported that poly (I:C)-induced TLR3 signalling is not inhibited by TGF-β1 in RAW264.7 cells [3] , our results showed that pre-treatment of TGF-β1 significantly inhibited IFNB1 expression induced by MyD88-independent TLR3 signalling 6 h after poly (I:C) treatment in primary peritoneal macrophages ( Fig. 7f ; Supplementary Fig. S6 ). However, the inhibitory effects of TGF-β1 on TLR3 signalling was decreased in SMAD6 knockdown primary macrophages, but not in SMURF1 or SMURF2 knockdown cells ( Fig. 7g ; Supplementary Fig. S6 ), indicating that TGF-β1-induced suppression of MyD88-independent TLR3 signalling may imply the presence of an independent process mediated by Smad6, but not by the Smad6–Smurf1 pathway. Collectively, our results suggest that MyD88 degradation by the Smad6–Smurf pathway is a crucial mechanism underlying TGF-β1-mediated suppression of MyD88-dependent TLR signalling pathways, including the TLR2 and TLR4 pathways. To maintain tissue homeostasis, inflammatory responses must be resolved by several mechanisms, including short half-lives of inflammation mediators and anti-inflammatory signals. Prolonged or excessive inflammation may cause the accumulation of a variety of cellular injuries such as DNA damage, eventually resulting in inflammation-related diseases such as cancer, atherosclerosis and obesity [35] , [36] , [37] , [38] . Here we define a distinct role of the anti-inflammatory TGF-β cytokine and provide insight into the molecular mechanisms behind the TGF-β1-induced ubiquitination and degradation of MyD88. Our novel findings are as follows. First, we have uncovered a new role for Smurf proteins in the TGF-β1 anti-inflammatory response, where they suppress pro-inflammatory signals via K48-linked polyubiquitination of the adaptor MyD88. The possible role of the Smurf1 protein in an anti-inflammation process is supported by a recent report about on Smurf1-mediated ubiquitination and degradation of TRAF family proteins [39] . Our findings add to the diverse roles of the Smurf proteins, which include their traditional role as antagonists of TGF-β/bone morphogenic protein signalling, and a more recently discovered role in planar cell polarity through the non-canonical Wnt signalling pathway [40] . Second, we provide further evidence for a distinct role of Smad6 from Smad7, although both are anti-inflammatory mediators. Previously, only Smad7 was found to be involved in the negative regulation of TNF-α signalling [5] . In this study, we found that TGF-β1-induced ubiquitin-mediated degradation of MyD88 is dependent on the presence of Smad6, but not Smad7. SMAD7 knockdown experiments by lentiviral infections in both primary peritoneal macrophages and CMT-93 epithelial cells did not show MyD88 ubiquitination and degradation on TGF-β1 treatment. Third, Smad6 is required to recruit Smurf1 to MyD88. In SMAD6 knockdown cells, the formation of MyD88-Smad6-Smurf1 was not observed and ectopic expression of Smad6 restored the recruitment of Smurf1 to MyD88. In contrast, Smurf2 does not directly bind to Smad6 but is involved in MyD88 degradation via interaction with Smurf1. In light of our results, and also the previous results, that Smurf1 interacts with Smurf2 (ref. 32 ), it is unclear why MyD88 degradation was observed in SMURF2 single knockdown cells. We speculate that the Smurf1 and Smurf2 proteins are likely in a single complex where they reciprocally influence the activity or stability of the other protein. Fourth, the TGF-β1 anti-inflammatory activity mediated by degradation of MyD88 by the Smad6–Smurf pathway is likely to be effective in other MyD88-dependent TLR signalling pathways, not only the TLR4 pathway. However, our finding that the TLR3 pathway is inhibited through a mechanism mediated by TGF-β1-induced Smad6, which is not the Smad6–Smurf pathway, is inconsistent with results by Naiki et al . [3] Interestingly, a recent report [41] suggests that TGF-β1 may inhibit MyD88-independent TLR3 signalling. Pellino-1 was identified as a binding partner of IKKɛ, and IKKɛ/TBK1 activated Pellino-1 in response to TLR3 and TLR4 agonists [41] . The IKKɛ/TBK1 complex, which is downstream of the adaptor TRIF in TLR3 signalling, acts as protein kinases that activate the IRF3 transcription factor, stimulating expression of the IFNB1 gene [17] , [42] . Because TGF-β1-induced Smad6 negatively regulates TLR4 signalling through direct binding to Pellino-1 (ref. 4 ), we speculate that TGF-β1 induces Smad6, and that the increased levels of Smad6 subsequently inhibit TLR3 signalling through disruption of IKKɛ/TBK1/Pellino-1 via binding to Pellino-1, but not through the Smad6–Smurf pathway. Finally, we provide evidence that TGF-β-mediated negative regulation of IL-1R/TLR signalling is accomplished through at least two distinct mechanisms. TGF-β1-induced Smad6 and Smad7 were reported to bind to the adaptor Pellino-1 to disrupt the IL-1R/TLR signalling complex IRAK1-IRAK4-Pellino-1-TRAF6 (refs 4 , 33 ). However, knockdown of PELI1 in CMT-93 cells did not prevent the ubiquitination and degradation of the MyD88 protein ( Supplementary Fig. S8 ), indicating that Pellino-1 is not involved in TGF-β1-induced ubiquitination and degradation of MyD88. Therefore, TGF-β-mediated anti-inflammatory activity suppressing the IL-1R/TLR pro-inflammatory signal appears to be accomplished through at least two distinct mechanisms, by targeting either MyD88 or Pellino-1 through the inhibitory Smads. In conclusion, we demonstrate that the TGF-β1-induced K48-linked ubiquitination and degradation of MyD88 driven by the Smad6–Smurf pathway is a novel mechanism that negatively regulates MyD88-dependent pro-inflammatory signalling. Thus, modulation of Smurf proteins, as well as Smad6, may be an important therapeutic strategy for the treatment of TLR4 or TLR2-related diseases. Plasmids The full-length MyD88 complementary DNA was cloned into the Bam HI and Eco RI sites of pcDNA3.1/His vector (Invitrogen), resulting in His-MyD88. Plasmids encoding different regions of the MyD88 protein (Flag-MyD88-N, Flag-MyD88-M, Flag-MyD88-C, Flag-MyD88-FL, Flag-MyD88-1/2L and Flag-MyD88-1/2R) were amplified from full-length His-MyD88 cDNA by PCR and subcloned into the Bam HI and Eco RI sites of the pCMV-Flag vector (Stratagene). Flag-Smad6-MH1-like, Flag-Smad6-Linker, Flag-Smad-MH2 and Flag-Smad6 FL were previously described [33] . The full-length Smad6 cDNA was cloned into the Bam HI and Not I sites of pSG5-2xHA, which contains 2 copies of the HA epitope. The full-length human Smurf1 cDNA was cloned into the Bgl II and Xho I sites of the pCMV-6xMyC vector, which contains 6 copies of the Myc epitope. The full-length human Smurf2 cDNA was cloned into the Eco RI and Hind III sites of the pCMV-Flag vector, and the Eco RI and Not I sites of the pSG5-2xHA vector. The plasmids expressing wild-type His-ubiquitin (His-Ubi), His-UbiK48, His-UbiK63, and His-Ubi7KR were provided by Dr Jaewhan Song (Yonsei University, Korea). In His-UbiK48, six lysine residues were mutated into arginine residues, except for lysine residue 48, whereas only lysine residue 63 was normal in His-UbiK63. All seven lysine residues of ubiquitin were mutated into arginines in His-Ubi7KR. The lysine to arginine MyD88 point mutants were generated using the QuikChange mutagenesis kit (Stratagene). Myc-Smurf1 C699A and HA-Smurf2 C695A were also constructed using the QuikChange mutagenesis kit. Sequences of PCR-generated portions of all constructs were verified by sequencing. Primer sequences for PCR are described in Supplementary Table S1 . The 5x NF-κB-Luc luciferase reporter plasmid was purchased from Clontech Laboratories. Reagents and cell culture Recombinant human TGF-β1 was obtained from R&D Systems. LPS ( Escherichia coli serotype O11:B4) and MG132 were purchased from Sigma. LTA was a gift of Dr Seung Hyun Han (Seoul National University, Korea). CMT-93 murine intestinal epithelial cells, human embryonic kidney 293 (HEK293) cells, and RAW264.7 macrophage cells were maintained in DMEM with 10% FBS (GIBCO–BRL). For isolation of peritoneal macrophages, 8-week-old C57BL/6 female mice were injected with 3 ml of 3% thioglycollate (Sigma). After 4 days, peritoneal cells were washed out with PBS and cultured at 37 °C in the presence of 5% CO 2 in DMEM supplemented with L-gluamine, antibiotics and 10% FBS. Animal protocols were approved by the Institutional animal care and use committee of the department of biological sciences, Sungkyunkwan university (Suwon, Korea). Construction of small hairpin RNAs and lentiviral infection The short hairpin RNA (shRNA) sequences specific for endogenous SMAD6 , SMURF1 , SMURF2 and MYD88 are described in Supplementary Table S2 . Lentiviruses expressing shRNAs specific for endogenous SMAD7 were previously described [4] , [5] . To generate shRNAs specific for endogenous SMAD6 , SMURF1 , SMURF2 and MYD88 , double-stranded oligomers containing restriction enzyme sites, a sense sequence, and a loop sequence with its antisense sequence were designed and cloned into Age I and Eco RI sites of the pLKO-puro vector (Clontech). Lentiviruses expressing each siRNA were produced by a lentiviral packaging system from Invitrogen. Lentivirus expressing mutant Serpin2 (mPAI-2) siRNA was used as a negative control for lentivirus infection [4] . SMAD6 and PELI1 knockdown CMT-93 cell lines The SMAD6 knockdown CMT-93 cells (CMT-93-si-S6) expressing a siRNA specific for endogenous SMAD6 , and the control CMT-93 cells with the pU6PL vector (CMT-93 wild type) were previously described [4] . To construct PELI1 knockdown CMT-93 cells (CMT-93-si-Pellino-1), 5′-AATATGGTGAACTCATTGTC-3′ was empirically selected as a target sequence for Pellino-1. A pair of oligomers containing restriction enzyme sites, a PELI1 sense sequence, and a loop sequence with its antisense sequence were produced and inserted into the Bam HI and Hind III sites of the pU6PL vector, generating the plasmid pU6PL-si-Pellino-1. Inserted sequences were verified by DNA sequencing. To generate PELI1 knockdown cell lines, pU6-si-Pellino-1 was transfected into CMT-93 cells, and subclones showing neomycin resistance were initially selected. Among the candidate subclones, reduction in Pellino-1 expression was verified by RT–PCR analysis. Antibodies and ubiquitination assays Mouse anti-HA (mAb: F-7, dilution ratio 1:1,000), rabbit anti-His (H-15, 1:1,000), mouse anti-c-Myc (mAb: 9E10, 1:1,000), goat anti-Smad7 (N-19, 1:2,000), rabbit anti-Smad7 (H-79, 1:2,000), rabbit anti-Smurf1 (H-60, 1:2,000), rabbit anti-Smurf2 (H50, 1:2,000) were purchased from Santa Cruz Biotechnology. Mouse anti-ubiquitin-HRP antibody (1:1,000) was purchased from Bio-Mall. Rabbit anti-MyD88 (1:4,000) and rabbit anti-Smad6 antibodies (1:4,000) were purchased from Cell Signaling. Mouse anti-Flag (M2, 1:5,000), rabbit anti-Flag (1:5,000) and anti-β-actin (1:5,000) antibodies were obtained from Sigma. Ubiquitination assays of endogenous or ectopically expressed MyD88 were performed as described [43] , [44] , [45] with minor modifications. Cells were transfected with the indicated plasmid, and subsequently treated with TGF-β1 in certain conditions. Cells were collected in 1 ml PBS containing 5 mM N-ethyl maleimide (NEM) and centrifuged at 800 g for 3 min. Non-covalent protein interactions were dissociated with 1% SDS and boiled for 10 min. Samples were diluted ten times with lysis buffer (PBS containing 0.5% Triton X-100, 20 mM HEPES (pH 7.4), 150 mM NaCl, 12.5 mM β-glycerol phosphate, 1.5 mM MgCl 2 , 10 mM NaF, 2 mM DTT, 1 mM NaOV, 2 mM EGTA, 1 mM PMSF, and protease inhibitor cocktail) and subsequently suspended by using a 1 ml syringe. The samples were cleared by centrifugation at 16,000 g for 10 min. For immunoprecipitation, lysates were incubated with protein A/G agarose beads and with anti-His antibody at 4 °C for 12 h. The beads were washed three times with lysis buffer and immunoprecipitates were separated from the beads by adding 2× sample buffer and were boiled and fractioned by SDS–PAGE. Immunoblot analysis was subsequently performed using the indicated antibodies. For ubiquitination assays of endogenous MyD88, SDS–PAGE-separated immunoprecipitates were transferred onto PVDF membranes. The membranes were denatured with denaturation buffer containing 6 M guanidine chloride, 20 mM Tris (pH 7.5), 100 mM PMSF, and 5 mM β-mercaptoethanol at 4 °C for 30 min and washed three times with PBST. The membranes were blocked with 5% BSA and incubated with anti-ubiquitin-HRP antibody. Transient transfection and reporter assay All plasmids were transiently transfected into HEK293 or CMT-93 cells using Effectene (Qiagen). Cells were treated for the indicated time with TGF-β1 (5 ng/ml) or treated with MG132 (5 μM) for 6 h followed by TGF-β1 (5 ng/ml) for 2 h. For certain experiments, cells were pre-treated with TGF-β1 (5 ng/ml) for 2 h before treatment of LPS (10 ng/ml), LTA (2 μg/ml), or poly (I:C) (5 μg/ml). Luciferase activity was normalized to β-galactosidase activity to adjust for variations in transfection efficiency. All experiments were independently repeated at least three times with similar results. Pull-down and ubiquitination assay by Ni-NTA columns Cells were collected in PBS buffer containing 5 mM NEM. Cells were resuspended in binding buffer (6 M guanidine HCl, 0.1 M Na 2 HPO 4 , 0.1 M NaH 2 PO 4 , 0.01 M Tris (pH 8.0), 10 mM β-mercaptoethanol, 5 mM NEM, 5 mM imidazole) and incubated with Ni-NTA agarose (Qiagen) at 4 °C for 12 h. The Ni-NTA agarose was sequentially washed with buffer A (6 M guanidine HCl, 0.1 M Na 2 HPO 4 , 0.1 M NaH 2 PO 4 , 0.01 M Tris (pH 8.0), 10 mM β-mercaptoethanol), buffer B (8 M Urea, 0.1 M Na 2 HPO 4 , 0.1 M NaH 2 PO 4 , 0.01 M Tris (pH 8.0), 10 mM β-mercaptoethanol), buffer C (8 M Urea, 0.1 M Na 2 HPO 4 , 0.1 M NaH 2 PO 4 , 0.01 M Tris (pH 6.3), 10 mM β-mercaptoethanol, 0.2% Triton X-100), and buffer D (8 M Urea, 0.1 M Na 2 HPO 4 , 0.1 M NaH 2 PO 4 , 0.01 M Tris (pH 6.3), 10 mM β-mercaptoethanol, 0.1% Triton X-100). The resulting Ni-NTA agarose was suspended in elution buffer (2× sample buffer, 0.72 M β-mercaptoethanol, 200 mM imidazole), incubated at room temperature for 20 min, and then boiled for 10 min. After brief centrifugation, samples were loaded into SDS–PAGE gels. Immunoblotting was performed using anti-Flag antibodies. Endogenous Smad6 was detected with anti-Smad6 antibody. Expression of the β-actin protein was used as a loading control. Immunoflourescence Cells were fixed in cold 4% paraformaldehyde for 30 min, and permeabilized in 0.25% Triton X-100 at room temperature for 2 min, followed by incubation with primary antibodies at 37 °C for 3 h. Anti-NF-κB p65 (1:300) antibody was used to detect NF-κB nuclear translocation. Anti-Flag (1:300), anti-HA (1:300) and anti-Myc (1:300) antibodies were used for detecting the co-localization of Flag-MyD88, HA-Smad6 and Myc-Smurf1. After five washes in PBS, coverslips were incubated at 37 °C for 3 h with the following secondary antibodies: Rhodamin-conjugated goat anti-rabbit IgG (1:500, for anti-NF-kB p65 and anti-Flag antibodies), FITC-conjugated goat anti-mouse IgG (1:500, for anti-Myc antibody), or Cy5-conjugated Rabbit anti-goat IgG (1:500, for anti-HA antibody). Coverslips were stained with DAPI (Santa Cruz) and mounted on a slide glass. Cells were examined with laser-scanning microscopy (Carl-Zeiss). Details of the immunoblot analysis, immunoprecipitation, RNA extraction, regular RT–PCR, quantitative real-time RT–PCR and ELISA are provided in the Supplementary Methods . How to cite this article: Lee, Y. S. et al . Smad6-specific recruitment of Smurf E3 ligases mediates TGF-β1-induced degradation of MyD88 in TLR4 signalling. Nat. Commun. 2:460 doi: 10.1038/ncomms1469 (2011).